Creation of a two-dimensional electron gas at an oxide interface on silicon In recent years, reversible control over metal-insulator transition has been shown, at the nanoscale, in a two-dimensional electron gas (2DEG) formed at the interface between two complex oxides. These materials have thus been suggested as possible platforms for developing ultrahigh-density oxide nanoelectronics. A prerequisite for the development of these new technologies is the integration with existing semiconductor electronics platforms. Here, we demonstrate room-temperature conductivity switching of 2DEG nanowires formed at atomically sharp LaAlO 3 /SrTiO 3 (LAO/STO) heterointerfaces grown directly on (001) Silicon (Si) substrates. The room-temperature electrical transport properties of LAO/STO heterointerfaces on Si are comparable with those formed from a SrTiO 3 bulk single crystal. The ability to form reversible conducting nanostructures directly on Si wafers opens new opportunities to incorporate ultrahigh-density oxide nanoelectronic memory and logic elements into well-established Si-based platforms. Heterointerfaces between different oxide layers can display remarkable electrical properties [1] that differ from either constituent, such as a two-dimensional electron gas (2DEG, refs 2 , 3 , 4 , 5 , 6 , 7 , 8 , 9 , 10 , 11 , 12 , 13 , 14 ) and interfacial superconductivity [15] . The discovery of a 2DEG (ref. 3 ) at the heterointerface between band insulators LaAlO 3 (LAO) and SrTiO 3 (STO) has launched many experimental [2] , [3] , [4] , [5] , [6] , [7] , [8] , [9] , [10] , [11] , [12] , [16] and theoretical [13] , [17] , [18] investigations of the fundamental origins and properties of this novel electronic state. Thiel et al . [7] reported non-volatile electrical control of a metal-insulator quantum phase transition in LAO/STO heterointerface at room temperature. At low temperatures, another electrical field-induced quantum phase transition, from insulating to superconducting, was observed [8] . Recently, Cen et al . [2] demonstrated nanoscale lateral confinement of a 2DEG at a LAO/STO heterointerface with an LAO thickness of 3 unit cells (uc) by using a conducting atomic force microscope (c-AFM) lithography technique. Metallic nanoislands, nanowires and transistors were constructed with characteristic dimensions approaching 1 nm, without the need for complex lithographic procedures [4] . Silicon (Si) is the most desirable platform for the development of multifunctional oxide-based nanoelectronic devices, including field-effect transistors and non-volatile memory elements, fashioned out of 2DEG channels [4] . Central to these challenges are the integration of an oxide nanoelectronic device with Si-based electronic circuits [19] , [20] and scaling to a commercially available and Si-compatible large wafer process. On the other hand, it was reported that the heterointerface between LAO and TiO 2 -terminated STO (TiO 2 -STO) exhibited a metallic 2DEG behaviour, whereas the heterointerface between LAO and SrO-terminated STO (SrO-STO) showed an insulating behaviour [3] , [6] . In addition, the transport properties of 2DEG at LAO/STO interfaces are strongly influenced by scattering at dislocation cores [10] . These indicate that a STO platform with a high crystalline quality and TiO 2 -single surface termination is critical for the fabrication of a novel oxide heterointerface exhibiting 2DEG behaviour. For these reasons, most previous studies on 2DEG at the heterointerface between different perovskite oxide layers have been achieved on STO bulk single crystal substrates having a well-defined TiO 2 -single termination and an atomically smooth surface [21] . Here, we demonstrate the reversible conductivity switching of a 2DEG with nanoscale dimension at the LAO/STO heterointerfaces directly on Si substrates by c-AFM lithography [2] . The processes of writing and erasing a conducting nanowire by c-AFM were reproducible and the electrical properties of LAO/STO heterointerfaces on Si were strongly influenced by the characteristics of the STO template, such as surface termination and defect density [10] . Improvement of surface properties of STO templates by post-annealing The oxide heterostructures for nanowriting experiments consist of epitaxial 3 uc LAO and 100-nm-thick STO templates on Si substrates. Epitaxial (001) STO templates of 100 nm thickness were grown on (001) Si substrates by molecular beam epitaxy. [22] The termination of epitaxial STO films was controlled by halting film growth at SrO and TiO 2 . Mixed-termination surfaces were also investigated. To improve the crystalline quality and surface morphology, STO templates on Si were annealed at 900 °C for 2 h in O 2 atmosphere [23] and compared with an as-grown STO template on Si. AFM images of TiO 2 -STO templates acquired before and after annealing demonstrate the importance of the annealing step. The as-grown TiO 2 -STO template shows many small islands on the surface ( Fig. 1a ), whereas the annealed TiO 2 -STO template exhibits an atomically smooth surface with larger islands because of the coarsening of small islands during high-temperature annealing ( Fig. 1b ). Both SrO- and uncontrolled-termination STO templates on Si also showed atomically smooth surfaces after annealing. 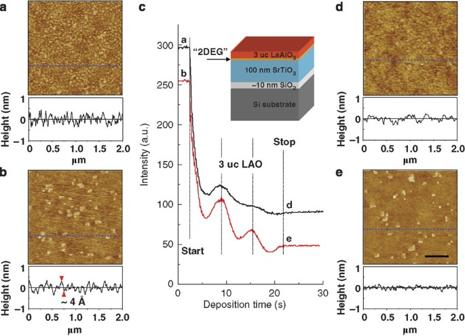Figure 1: Growth of LAO films on STO/Si substrates. AFM images of 100-nm-thick epitaxial (001) TiO2-STO films on (001) Si substrates (a) before and (b) after annealing. (c) RHEED intensity oscillations of LAO films on as-grown (black line) and annealed (red line) TiO2-STO/Si substrates. The vertical dot lines indicate the growth time of LAO unit-cell layer. Inset shows the schematic diagram of the LAO/STO heterostructure on Si substrate. The LAO/STO heterointerfaces were atomically controlled, either (LaO)+-(TiO2)0or (AlO2)−-(SrO)0. AFM images of 3 uc LAO films on (d) as-grown and (e) annealed TiO2-STO/Si. The dimension of the scale bar is 500 μm. The bottom panels of AFM images correspond to the cross-sectional profiles of blue dot lines in AFM images. Figure 1: Growth of LAO films on STO/Si substrates. AFM images of 100-nm-thick epitaxial (001) TiO 2 -STO films on (001) Si substrates ( a ) before and ( b ) after annealing. ( c ) RHEED intensity oscillations of LAO films on as-grown (black line) and annealed (red line) TiO 2 -STO/Si substrates. The vertical dot lines indicate the growth time of LAO unit-cell layer. Inset shows the schematic diagram of the LAO/STO heterostructure on Si substrate. The LAO/STO heterointerfaces were atomically controlled, either (LaO) + -(TiO 2 ) 0 or (AlO 2 ) − -(SrO) 0 . AFM images of 3 uc LAO films on ( d ) as-grown and ( e ) annealed TiO 2 -STO/Si. The dimension of the scale bar is 500 μm. The bottom panels of AFM images correspond to the cross-sectional profiles of blue dot lines in AFM images. Full size image The LAO films of varying thickness were grown epitaxially on STO/Si substrates by pulsed-laser deposition (PLD) with in situ high-pressure reflection high-energy electron diffraction (RHEED) [24] . During growth, LAO films on annealed STO/Si exhibited clear RHEED intensity oscillations ( Fig. 1c ), regardless of surface termination. In contrast, well-defined RHEED oscillations were not observed during growth on as-grown STO/Si. From this result, it can be concluded that the LAO film on the annealed STO/Si substrate was well grown in a layer-by-layer mode. This result also supports that high-temperature post-annealing improves the morphology of the STO templates, as shown in Figure 1a,b . After deposition, the epitaxial LAO films also showed atomically smooth surfaces, as shown in Figure 1d,e . Interface and defect structures of the LAO/STO heterostructure on Si To investigate the interface and defect structures of the LAO/STO heterostructure on Si, 5-nm-thick LAO films on as-grown and annealed TiO 2 -STO/Si were studied by transmission electron microscopy (TEM). 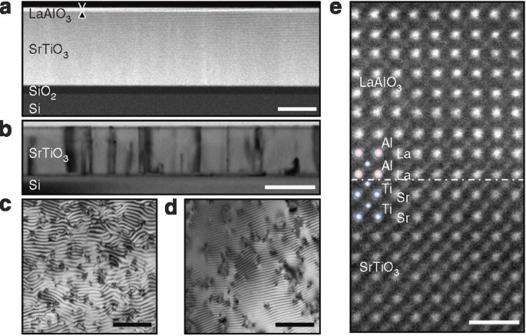Figure 2: TEM investigation of the LAO/STO heterointerface on Si. (a) A cross-sectional high-angle annular dark field (HAADF) image of a 5-nm-thick LAO/annealed TiO2-STO heterostructure grown on Si. Arrows indicate the thickness of the LAO layer. The scale bar corresponds to 50 nm. (b) A cross-sectional bright-field TEM image of the same sample showing the existence of threading dislocations in the STO layer. Planar-view TEM images of (c) as-grown and (d) annealed STO films showing moiré patterns. The scale bars inb,canddcorrespond to 100 nm. (e) A high-resolution HAADF image showing an atomically sharp interface between LAO film and annealed TiO2-STO on Si. The dimension of the scale bar is 1 nm. Figure 2a shows a cross-sectional high-angle annular dark field image of the heterostructure grown on annealed TiO 2 -STO/Si. After annealing, the dislocation density of the STO template decreased, but many dislocation lines were still observed because of the lattice mismatch between STO and Si ( Fig. 2b ). Figure 2a also shows that each layer of the heterostructure has a uniform thickness. Planar-view TEM studies of both as-grown and annealed TiO 2 -STO grown on Si show that the density of threading dislocations was reduced from 1.5 × 10 11 to 8.9 × 10 10 cm −2 by annealing. Moiré fringes can be observed in the thick areas of the planar-view samples because of the overlap between STO and Si substrate ( Fig. 2c,d ). Uniform straight fringes are expected if a perfect STO thin layer is overlapped with a single crystal Si substrate. Moiré fringes show discontinuities at threading dislocations (which have a Burgers vector of either [100] or [110] of STO) and change in spacing and orientation due to the lattice distortion induced by dislocations in STO. In as-grown STO films, threading dislocations show a uniform distribution and a serious lattice distortion is observed ( Fig. 2c ). In contrast, the dislocations in the annealed sample show a relatively low density and a non-uniform distribution, which results in large regions with almost perfect structure and orientation surrounded by 'boundaries' formed by dislocations ( Fig. 2d ). This study reveals that the structural quality of STO films was improved by thermal annealing, although the density of threading dislocations is reduced only by 30%. In addition, the atomic structure of the LAO/STO interface was studied by subangstrom scanning TEM. The high-angle annular dark field image in Figure 2e shows that LAO film is coherently grown on an annealed TiO 2 -STO template with an atomically sharp interface (the positions of atomic columns are indicated by circles). Figure 2: TEM investigation of the LAO/STO heterointerface on Si. ( a ) A cross-sectional high-angle annular dark field (HAADF) image of a 5-nm-thick LAO/annealed TiO 2 -STO heterostructure grown on Si. Arrows indicate the thickness of the LAO layer. The scale bar corresponds to 50 nm. ( b ) A cross-sectional bright-field TEM image of the same sample showing the existence of threading dislocations in the STO layer. Planar-view TEM images of ( c ) as-grown and ( d ) annealed STO films showing moiré patterns. The scale bars in b , c and d correspond to 100 nm. ( e ) A high-resolution HAADF image showing an atomically sharp interface between LAO film and annealed TiO 2 -STO on Si. The dimension of the scale bar is 1 nm. 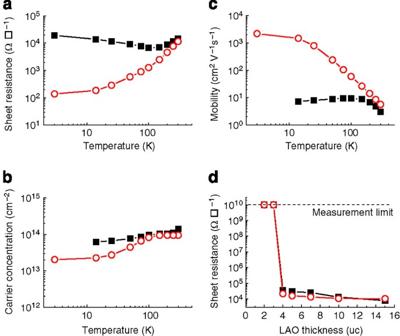Figure 3: Electrical transport properties of LAO/STO heterointerface on Si. Temperature dependence of (a) sheet resistance, (b) carrier concentration and (c) mobility of the heterointerface between unpatterned 10 uc LAO and TiO2-STO on Si (black squares). The STO layer on the Si substrate without the LAO layer showed highly insulating behaviour, indicating that the measured transport properties of LAO/STO on Si originated only from 2DEG. For comparison, the electrical transport properties of unpatterned 10 uc LAO on STO single crystal were also measured (red circles). (d) LAO thickness dependence of sheet resistance of unpatterned LAO/STO heterointerface on Si. Full size image Electrical transport properties of LAO/STO heterointerface on Si The temperature dependence of the sheet resistance, carrier concentration and mobility of an unpatterned heterointerface between 10 uc LAO and annealed TiO 2 -STO on Si by van der Pauw method are shown in Figure 3a–c . The room-temperature properties are comparable with those for heterointerfaces between LAO and STO bulk single crystals [3] , [25] . Although the low-temperature mobility is much lower than that of the LAO/STO single crystal, presumably because of sensitivity to the defect structure of the heterointerface, we believe that the 2DEG at the LAO/STO heterointerface on Si could be useful for room-temperature nanoelectronic devices. We compared the room-temperature thickness-dependent electrical properties of unpatterned LAO/STO on Si and LAO on STO bulk single crystal grown under identical conditions ( Fig. 3d (sheet resistance) and Supplementary Fig. S1 (carrier concentration and mobility)). Both sets of samples showed the same 4 uc critical thickness. The only apparent differences were a lower mobility and somewhat larger sample-to-sample variation for LAO/STO on Si. We have also measured the electrical properties of the STO layer on Si. It showed insulating behaviour relative to the interfacial 2DEG for LAO thicknesses above the critical thickness. This supports the conclusion that our measured transport properties of unpatterned LAO/STO on Si above the critical thickness originated only from the 2DEG and not the Si substrate. The bare Si substrate was determined to be of p -type, with a room-temperature mobility μ ~350 cm 2 V −1 s −1 and carrier concentration n ~0.8 × 10 15 cm −3 , significantly different from the electrical properties of the interfacial 2DEG for LAO/STO on Si (see Supplementary Fig. S2 ). Figure 3: Electrical transport properties of LAO/STO heterointerface on Si. Temperature dependence of ( a ) sheet resistance, ( b ) carrier concentration and ( c ) mobility of the heterointerface between unpatterned 10 uc LAO and TiO 2 -STO on Si (black squares). The STO layer on the Si substrate without the LAO layer showed highly insulating behaviour, indicating that the measured transport properties of LAO/STO on Si originated only from 2DEG. For comparison, the electrical transport properties of unpatterned 10 uc LAO on STO single crystal were also measured (red circles). ( d ) LAO thickness dependence of sheet resistance of unpatterned LAO/STO heterointerface on Si. Full size image Generation of 2DEG nanowires using c-AFM Nanowriting experiments were carried out on 3 uc LAO/STO heterointerfaces on Si, a thickness just below the critical thickness for the onset of conduction. The heterointerface conductance is modulated locally using a c-AFM tip that is scanned in contact mode across the LAO surface [7] . A conducting 2DEG nanowire is created by scanning the c-AFM tip along the x -axis with a tip potential of V tip =+4 V ( Fig. 4a ). When the c-AFM tip reaches from one to the other electrode, an abrupt jump in current is observed ( Fig. 4b ). 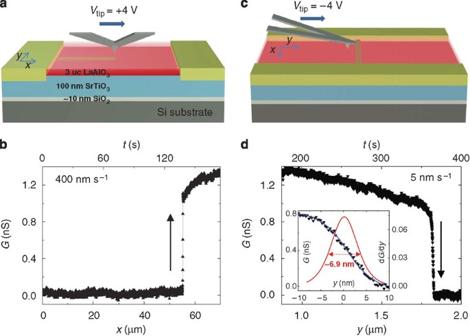Figure 4: Processes of writing and erasing a nanowire at the LAO/TiO2-STO heterointerface on Si. (a) Schematic diagram of the 'writing' process used to generate conducting nanostructures at the LAO/TiO2-STO heterointerface. (b) Electrical conductance between two electrodes during c-AFM writing withVtip=+4 V. As the c-AFM tip reaches the second electrode, the conductance increases abruptly. The c-AFM tip travels along thex-direction as noted in the figure, with a speed of 400 nm/s relative to the structure. (c) Schematic diagram of the 'erasing' process by cutting the nanowire generated in the writing process. (d) As the c-AFM tip biased at −4 V scans cross the nanowire, the conductance decreases drastically. The c-AFM tip travels at a speed of 10 nm s−1along they-direction, as indicated. The width of the nanowire presented in the inset is quantified by fitting the erase curve with a functionG(x)=G0−G1tanh(x/h), with the following best-fit parameters:G0=0.40 nS,G1=0.44 nS andh=6.0 nm. The deconvolved differential conductance (dG/dx)*−1is shown in red and has a half-width maximum of 6.9 nm (+4 V wire). After writing the nanowire, the tip is repositioned as shown in Figure 4c , biased negatively ( V tip =−4 V) and scanned slowly along the y- direction. When the tip reaches the nanowire, the conductance abruptly reaches zero again ( Fig. 4d ). An analysis of the sharpness of the cutting profile provides a measure of the nanowire width [2] , which in this case is w ~6.9 nm. The oxide nanostructures created on Si substrates display a resistivity comparable with those reported previously for STO single crystals. The two-dimensional sheet resistance can be calculated as R = w / lσ ≈1.9 × 10 5 Ω □ −1 , where w ≈6.9 nm, l =30 μm and σ =1.2 nS. In this measurement, parallel leakage current through SiO 2 to Si was subtracted (see Supplementary Fig. S3 ). The measured sheet resistance of an unpatterned sample with 4 uc LAO (just above the critical thickness) is ~4 × 10 4 Ω □ −1 . Figure 4: Processes of writing and erasing a nanowire at the LAO/TiO 2 -STO heterointerface on Si. ( a ) Schematic diagram of the 'writing' process used to generate conducting nanostructures at the LAO/TiO 2 -STO heterointerface. ( b ) Electrical conductance between two electrodes during c-AFM writing with V tip =+4 V. As the c-AFM tip reaches the second electrode, the conductance increases abruptly. The c-AFM tip travels along the x -direction as noted in the figure, with a speed of 400 nm/s relative to the structure. ( c ) Schematic diagram of the 'erasing' process by cutting the nanowire generated in the writing process. ( d ) As the c-AFM tip biased at −4 V scans cross the nanowire, the conductance decreases drastically. The c-AFM tip travels at a speed of 10 nm s −1 along the y -direction, as indicated. The width of the nanowire presented in the inset is quantified by fitting the erase curve with a function G ( x )= G 0 − G 1 tanh( x / h ), with the following best-fit parameters: G 0 =0.40 nS, G 1 =0.44 nS and h =6.0 nm. The deconvolved differential conductance (d G /d x )* −1 is shown in red and has a half-width maximum of 6.9 nm (+4 V wire). Full size image Multiple write and erase tests were conducted and the results were consistent with the data presented in Figure 4 . In addition, the writing and erasing of data for another set of electrodes showed similar behaviour. The minimum voltage required for creating a nanowire was 2.5 V, slightly smaller than that for 3 uc LAO on TiO 2 -terminated bulk STO. The existence of a conducting backplane (the Si substrate) may help with the writing process when the heterointerface is initially highly insulating. In addition, the width of a typical wire written with a +6 V c-AFM tip bias is comparable with the width of a wire written with V tip =+10 V on a 3 uc LAO/STO (ref. 2 ). 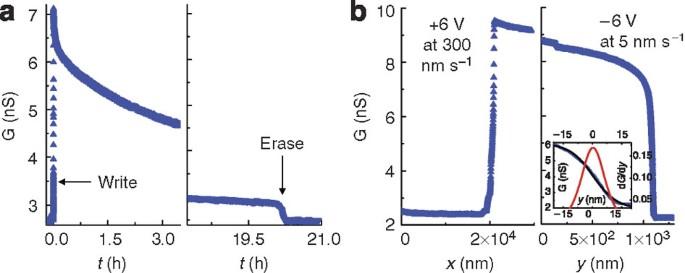Figure 5: Time decay for conductance of a nanowire. (a) Resilience of a nanowire written with a +6 V AFM tip bias and 300 nm s−1speed and kept overnight in the dark. The conductance decays exponentially at first and then linear over ~18 h. (b) The change in conductance for a +6 V write and −6 V erase nanowire and the calculated width as discussed in the main text. The width of the nanowire is quantified by fitting the erase curve with a functionG(x)=G0−G1tanh(x/h) with the following best-fit parameters:G0=3.8 nS,G1=0.68 nS andh=10.9 nm. The deconvolved differential conductance (dG/dx)*−1is plotted in red and has a full width at maximumy=9.7 nm. Electrical properties of 2DEG nanowires Figure 5 shows the increase in conductance for a nanowire written with an AFM tip bias of +6 V. Before writing the wire, the area around the used electrodes is scanned with a positive bias of 6 V; in this way a set of 'virtual electrodes' is created. The nanowire is written by scanning the AFM tip on the surface at a constant speed of 300 nm s −1 starting from the first gold electrode and ending on the second electrode as shown in Figure 4a,c . The wire was kept in darkness for almost 18 h before erasing. The non-exponential decay in atmospheric conditions ( Fig. 5a ) is comparable with that observed for LAO/STO heterostructures not grown on Si. The conductance of the wire written with V tip =+6 V ( Fig. 5b ) is significantly larger than for V tip =+4 V, again in qualitative agreement with experiments conducted on LAO/STO heterostructures. Figure 5: Time decay for conductance of a nanowire. ( a ) Resilience of a nanowire written with a +6 V AFM tip bias and 300 nm s −1 speed and kept overnight in the dark. The conductance decays exponentially at first and then linear over ~18 h. ( b ) The change in conductance for a +6 V write and −6 V erase nanowire and the calculated width as discussed in the main text. The width of the nanowire is quantified by fitting the erase curve with a function G ( x )= G 0 − G 1 tanh( x / h ) with the following best-fit parameters: G 0 =3.8 nS, G 1 =0.68 nS and h =10.9 nm. The deconvolved differential conductance (d G /d x )* −1 is plotted in red and has a full width at maximum y= 9.7 nm. Full size image We also investigated the nanowriting capabilities of the heterointerfaces between 3 uc LAO and STO templates with SrO- or uncontrolled-termination on Si substrates. However, neither of these heterointerfaces exhibited conductivity switching behaviour ( Table 1 ). In particular, we found that even the heterointerface between LAO on as-grown TiO 2 -STO/Si did not exhibit conductivity switching behaviour. We assume that this result is due to the defective surface of the as-grown STO template on Si. It is well known that as-grown oxide thin films have many defects such as dislocations, as well as many small islands ( Fig. 1a ). Therefore, such defects of the as-grown STO template likely hinder the formation of a 2DEG with nanoscale dimensions at the LAO/STO heterointerface. In contrast, the annealed STO template [23] has a relatively lower dislocation density through the annihilation of dislocations with contrary Burgers vectors and the dissociation of two whole dislocations into partial dislocations during high-temperature post-annealing [26] . In addition, the coarsening of small islands during post-annealing ( Fig. 1b ) results in a more well-defined (smoother) surface of STO template compared with that of the as-grown one because of the annihilation and redistribution of threading dislocations, as described in the previous section. Numerous nanowriting and conductivity switching experiments with heterointerfaces between LAO and STO bulk single crystals demonstrate a much higher sensitivity to the interface quality, such as defects, substrate quality and LAO film quality, compared with macroscopic transport measurements taken on conducting 2DEG layers grown on relatively thick LAO layers (that is, above 4 uc critical thickness). Therefore, it could be possible that the generation of a rewritable 2DEG nanowire only at the heterointerface between LAO and annealed TiO 2 -STO/Si is attributed not only to the TiO 2 -single surface termination but also to the low defect density of the annealed quasi-single-crystal STO template. Another possibility is that imperfect TiO 2 termination of thick films becomes tolerable as long as the conducting regions form a percolating network (see Supplementary Table S1 and Supplementary Figs S4 , S5 , S6 , S7 ). In quasi-one-dimensional structures, a single patch of SrO-terminated STO is sufficient to halt conduction. Table 1 Nanowriting capabilities of the heterointerfaces between 3 uc LAO and various STO templates on Si substrates. Full size table In summary, we have demonstrated for the first time the generation and conductivity switching of a 2DEG nanowire at an atomically sharp and coherent LAO/STO heterointerface grown directly on Si. Reversible conductivity switching of nanowires generated at the LAO/STO heterointerface directly on Si opens the possibility of the integration with Si for a variety of ultrahigh-density nanoelectronics applications. Growth of LAO/STO heterostructures on Si Epitaxial (001) STO thin films of 100 nm thickness were grown as template layers on 8-inch diameter (001) Si wafers by molecular beam epitaxy. The STO templates have different surface terminations, such as TiO 2 -, SrO- and uncontrolled-termination. The STO templates were annealed in a tube furnace under an oxygen atmosphere at 900 °C for 2 h. After annealing, the STO templates showed (002) rocking curve full-width at half-maximum of ~0.006°, which is much narrower than that of STO bulk single crystals [23] . Epitaxial thin films (3 uc) of LAO were deposited on the top of STO/Si substrates at 650 °C in an O 2 pressure of 1×10 −3 mbar by PLD. The PLD uses a KrF excimer laser (wavelength, λ =248 nm). The laser energy density is 2 J cm −2 . During the growth of LAO thin films, film thickness was controlled by in situ RHEED. The growth rate of LAO films is ~25 pulses per uc. After deposition, the LAO thin films were cooled down in O 2 pressure of 1×10 −3 mbar. Nanowire writing by c-AFM To measure the electrical conductivity of the heterointerface between 3 uc LAO and STO grown on Si substrates, electrical contacts to the 2DEG were made. Low-resistance contacts to the 2DEG heterointerface are created by a combination of Ar + milling (~25 nm deep) using a Commonwealth Scientific Ion beam etching system, followed by Ti/Au sputtering. First, a 2-nm Ti layer is sputter-deposited in order to create a good adhesion between the STO and Au, followed by ~23 nm of Au. Au wires are further bonded from the electrodes to a chip carrier. The nanowire writing is carried out using an Asylum MFP-3D AFM (Asylum) in contact mode. During scanning, a voltage, V tip , is applied to the tip, while the bottom Si substrate is held at ground level. Simultaneously, a small bias V 0 =0.1 V is applied to the left electrode, and the current is monitored at the right electrode, which is held at virtual ground level, using a femtoammeter. As with LAO/STO heterointerfaces not grown on Si substrates [1] , the 'writing' process ( V tip >0) locally switches the heterointerface to a conducting state, whereas the 'erasing' process ( V tip <0) locally restores the heterointerface to an insulating state. Electrical measurements were taken at room temperature in a dark environment to suppress carrier photoexcitation [1] in STO (bandgap ~3.2 eV). The writing and erasing of nanowires are reproducible at a given writing voltage. Leakage to the Si substrate through SiO 2 The current–voltage ( I–V ) characteristics measured between the two electrodes before and after writing a nanowire are shown in Supplementary Figure S3a . There is a significant nonlinear background before writing due to leakage to the Si substrate through the SiO 2 layer. Assuming that the nanowire produces a parallel conductance channel, the two curves may be subtracted to yield the I–V curve for the nanowire ( Supplementary Fig. S3b ). The residual nonlinearity observed is also attributed to direct coupling of the nanowire to the Si substrate. Increasing the thickness of the SiO 2 layer may help to reduce this leakage current, which is strongly asymmetric with applied voltage. Conductivity of LAO/STO/Si for various thicknesses of LAO The conductivity of a series of LAO films with varying thickness deposited on STO/Si was measured using a 'picoprobe' setup (GGB Industries). Two-terminal measurements were taken by contacting Au electrodes with the picoprobe sensors. The same electrode pattern was used for each sample in the series, and the electrical contacts were all made in a parallel process, as shown in Supplementary Figure S4 . The distance between the two picoprobes was constant for all measured samples. A matrix of 12 samples was investigated, corresponding to thicknesses 3, 4, 5 and 10 uc, and to three terminations: as-grown TiO 2 , annealed TiO 2 and annealed SrO. The I–V characteristics for these structures were measured at low voltages (−0.5 V< V <0.5 V) and conductance was calculated over a range for which the I–V curves were found to be linear (−0.2 V< V <0.2 V). All measurements have been taken using the same picoprobe setup as for the first thickness series. A summary of the conductance is presented in Supplementary Table S1 , and the curves are shown in Supplementary Figures S5–S7 . In the case of 3 uc LAO, only the heterointerface between LAO on annealed TiO 2 -STO was insulating before writing and writable. From all LAO/STO heterostructures, it is observed that there is a high increase in G between 3 uc and 4 uc before writing, which corresponds to the insulating-to-conducting transition seen before on LAO/STO bulk. The 5 uc and 10 uc heterostructures are highly conducting (ohmic) at the interface. The experiments show a clear transition from insulating to conducting interfaces as a function of thickness. However, it is interesting that the SrO-terminated samples also show a significant increase in conductance that approaches ~5% of the value for the TiO 2 -terminated samples at the largest thickness of 10 uc LAO. It is possible that SrO-terminated samples are not 100% terminated as SrO, but have residual (~5%) TiO 2 -terminated islands, which can contribute to the conduction at the interface through something similar to a percolation. However, we would be unable to write nanowires because those islands would not be percolating in one dimension. How to cite this article: Park, J.W. et al . Creation of a two-dimensional electron gas at an oxide interface on silicon. Nat. Commun. 1:94 doi: 10.1038/ncomms1096 (2010).